Identification of a novel salt tolerance gene in wild soybean by whole-genome sequencing Using a whole-genome-sequencing approach to explore germplasm resources can serve as an important strategy for crop improvement, especially in investigating wild accessions that may contain useful genetic resources that have been lost during the domestication process. Here we sequence and assemble a draft genome of wild soybean and construct a recombinant inbred population for genotyping-by-sequencing and phenotypic analyses to identify multiple QTLs relevant to traits of interest in agriculture. We use a combination of de novo sequencing data from this work and our previous germplasm re-sequencing data to identify a novel ion transporter gene, GmCHX1 , and relate its sequence alterations to salt tolerance. Rapid gain-of-function tests show the protective effects of GmCHX1 towards salt stress. This combination of whole-genome de novo sequencing, high-density-marker QTL mapping by re-sequencing and functional analyses can serve as an effective strategy to unveil novel genomic information in wild soybean to facilitate crop improvement. Advances in next-generation sequencing have driven a revolution in genomic analyses and their use for crop improvement, which is essential given the rapidly growing human population. There are several whole-genome-sequencing projects for major crops aiming to unveil novel insights in genomic evolution and diversity, including the effects of domestication and human selection [1] , [2] , [3] , and to apply whole-genome-sequencing data to actual crop improvement programmes. The genomic information in wild accessions complemented with detailed studies, and characterizations of genetic populations can help identify useful quantitative trait loci (QTLs) and candidate causal genes, some of which have already been successfully introgressed into cultivated accessions, for example, rice [4] , maize [5] and wheat [3] , for crop improvement. Soybean was domesticated in China ~6,000–9,000 years ago [6] , and, due to bottlenecks and human selection, cultivated soybeans have much lower genetic diversity than their wild counterparts [2] , [7] . This reduced variation has potentially resulted in the loss of some genes important for the adaptation to different environments. Wild soybeans that exhibit a high allelic diversity may therefore be a resource for genes for adapting to certain environmental conditions to be re-introduced into domesticated soybeans via breeding. This can be done since there is no reproductive barrier between wild and cultivated soybeans. Here we formulate a strategy to combine the whole-genome-sequencing approaches with de novo sequencing of a wild soybean genome and construction of genotyping-by-sequencing-based genetic map using a recombinant inbred (RI) population to assist in the genetic studies of important QTLs in the wild soybean genome. Further analyses with reference to the previously obtained re-sequencing data of germplasms [2] help in identifying GmCHX1 , a candidate causal gene for salt tolerance. 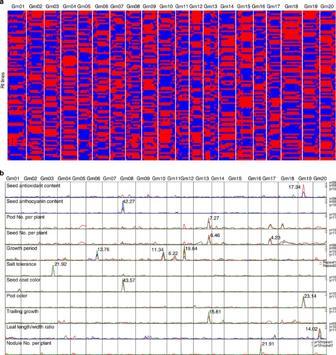Figure 1: QTL identification using bin map of a RI population. (a) Recombinant bin map of a core panel of 96 RI lines. Red and blue indicate parental genotypes from W05 and C08, respectively. (b) LOD score distribution of 11 agronomic traits with major QTLs. Maximum LOD score of each major QTL is indicated next to the peak. Different line colours indicate data collected in different years (yr08, 2008; yr09, 2009; yr10, 2010; yr11, 2011; and yr12, 2012). De novo assembly and annotation of a wild soybean genome We performed whole-genome de novo sequencing ( Supplementary Table 1 ) on W05, a wild soybean accession from China that our group previously characterized as having high tolerance to salt and is genetically and phylogenetically distinct from cultivated soybeans [2] . Its genome size is estimated at 1.17 Gb by K-mer statistics ( Supplementary Fig. 1 ), which is close to the estimated 1.12 Gb size of the cultivated soybean genome Williams 82 (ref. 8 ). 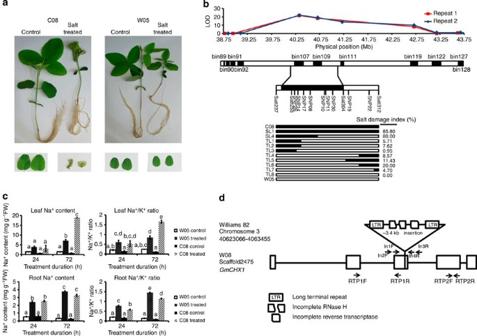Figure 2: Identification of a putative causal gene in the salt tolerance locus. (a) W05 exhibits a higher salt tolerance than C08. Bottom photos: primary leaves. (b) A 978-Kb salt tolerance locus is first identified by LOD score (upper panel), and narrowed down to a 388-Kb region using SNP and simple sequence repeat markers (middle panel) and extreme groups (lower panel). SL, sensitive line; TL, tolerant line. (c) W05 accumulates less Na+in the leaves than C08 72 h after NaCl treatment.N=4. Error bars=s.e.m.,P<0.05. (d) Gene structure ofGmCHX1in W05 and Williams 82. Arrows indicate primer positions for insertion and real-time PCR studies. FW, fresh weight. SOAPdenovo [9] software is used to build a 868-Mb assembly with sequencing reads ( Table 1 and Supplementary Table 2 ). The 3,281 largest scaffolds represent 90% of the assembled genome. 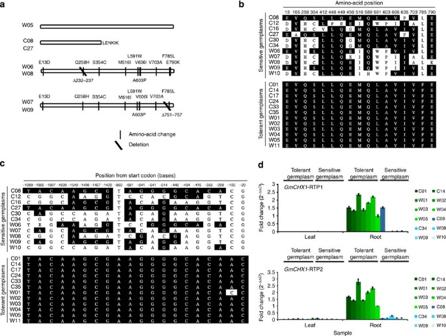Figure 3: TheGmCHX1gene is conserved among salt-tolerant soybean germplasms. (a) Structural variations in theGmCHX1coding region of salt-sensitive germplasms, with salt-tolerant W05 as comparison. (b) SNP analyses and multiple amino-acid sequence alignments of theGmCHX1coding region from different soybean germplasms. X denotes ambiguous amino acid due to low coverage of re-sequencing data. Black indicates conserved residues. (c) SNP analyses and multiple alignments of a 2-Kb promoter region ofGmCHX1from different soybean germplasms. Conserved bases are highlighted in black. R=G/A, Y=T/C. (d) Expression study ofGmCHX1in soybean germplasms. Real-time PCR of theGmCHX1gene using primers specific to regions upstream (upper panel; for tolerant lines and C08) or downstream (lower panel; for all germplasms) referenced to the retrotransposon insertion site in C08, using RNA from salt-tolerant (green bars) and salt-sensitive germplasms (blue bars).N=3. Error bar=s.e.m. More than 94% of the 742,658,772 cleaned reads from short insertion size libraries can be mapped to the 868-Mb genome, with 82% exhibiting proper pair-end relationships ( Supplementary Table 3 ). Table 1 Draft genome assembly and annotation of the wild soybean accession W05. Full size table Wild soybean genes are annotated using a combined gene model prediction strategy, integrating ab initio modelling, homology searching, expression-sequence tags and also using RNA-Seq data from transcriptomes generated for this project (trifoliate and primary leaves, and roots of young W05 seedlings; Supplementary Tables 4 and 5 ). To assess our annotation, we perform de novo assembly of the transcriptome raw data using Trinity [10] , and find a match for the majority of the assembled Trinity contigs in the annotated genome ( Supplementary Table 6 ). The Core Eukaryotic Genes Mapping Approach [11] further shows that the W05 (wild; this work) and Williams 82 (cultivated; [8] ) genomes are 86.7% and 90.3% complete, respectively ( Supplementary Table 7 ). (See Supplementary Figs 2 and 3 and Supplementary Tables 8 and 9 for detailed annotation information of the W05 genome.) RI population re-sequencing We construct a RI population by crossing the de novo -sequenced W05 with the re-sequenced cultivated soybean accession C08, a close relative of Williams 82, which has phenotypes different from those of W05 ( Supplementary Table 10 ). A core panel of 96 RI lines is selected for ~1 × depth low-level whole-genome re-sequencing ( Supplementary Table 11 ). After filtering, we identify 1,798,504 high-quality single-nucleotide polymorphisms (SNPs) that are distributed preferentially in the gene-harboring chromosome distal ends ( Supplementary Fig. 4 ) owing to the low frequency of meiotic recombinant events at the peri-centrimeric regions [12] . Heterozygosity of each RI line is low, reflecting the successful construction of a highly homozygous RI population ( Supplementary Table 11 ). Recombinant event determination We generate a bin map and determine the recombinant breakpoints of this RI population using the Maximum Parsimonious Inference of Recombination package [13] . Two thousand seven hundred and fifty-seven bin markers along the 20 chromosomes are identified, with their physical coordinates referenced to the Williams 82 genome (assembly version Glyma1.1) ( Fig. 1 and Supplementary Data 1 ). The total genetic length of this bin map is 2,992.0 cM in the Kosambi mapping function, with a mean interval between markers of 0.94 cM and an average physical bin length of 306.0 Kb. More than 60% of the recombinant breakpoints are located at the chromosome distal ends, consistent with a recent report [14] . Traditional simple sequence repeat markers are used to verify the quality and accuracy of the bin map. More than 94% of the PCR bands from experimental screening (total=61,856) share the same genotype with the corresponding bins. Figure 1: QTL identification using bin map of a RI population. ( a ) Recombinant bin map of a core panel of 96 RI lines. Red and blue indicate parental genotypes from W05 and C08, respectively. ( b ) LOD score distribution of 11 agronomic traits with major QTLs. Maximum LOD score of each major QTL is indicated next to the peak. Different line colours indicate data collected in different years (yr08, 2008; yr09, 2009; yr10, 2010; yr11, 2011; and yr12, 2012). Full size image High-density-marker QTL mapping of soybean traits We record 18 agronomic traits from the core panel RI lines and the two parents from different years ( Supplementary Table 10 and Supplementary Fig. 5 ). Most of the phenotypic data are quantitative and exhibit a normal distribution ( Supplementary Fig. 5 ). No major QTLs are found for seed oil content, seed protein content, 100-seed weight, leaf area, plant height, node number and branch number. However, we identify 15 major QTLs for 11 other traits from the high-density marker QTL map using QTLCartographer ( http://statgen.ncsu.edu/qtlcart/ ) ( Table 2 ). Sharp peaks in the log-of-odds (LOD) score curves for each QTL are obtained, spanning 11 of the 20 chromosomes ( Fig. 1b ). The LOD score cutoff for QTL identification ranges from 3.80 to 7.60, whereas the maximum LOD score for each trait ranges from 4.20 to 43.60. The identified QTLs occupy a physical length of 176 Kb to 1.28 Mb (average: 682.0 Kb; median: 601.6 Kb), with the genetic distances ranging from 0.5 to 7.9 cM (average 2.4 cM; median: 2.0 cM). For all mapped traits, the LOD score distributions calculated from trait data collected in different years are generally consistent ( Fig. 1b ). We map six QTLs for five of the 11 traits to genomic positions that coincide with QTLs in previously published reports ( Table 2 and Supplementary Table 12 ), providing support for the accuracy of this map. We identify nine new QTLs for seven traits, including total seed antioxidant content, seed anthocyanin content, pod number per plant, seed number per plant, growth period, pod colour and trailing growth ( Table 2 and Supplementary Table 12 ). Table 2 Major QTLs identified. Full size table We also examine the relationship among different QTLs. Three QTL clusters are identified on Chr08, Chr13 and Chr19 ( Fig. 1 and Table 2 ). Statistically significant correlations are observed among phenotypic characteristics mapped onto the same QTL cluster ( Supplementary Table 13 ). Cluster 1 on Chr08 contains QTLs for two closely related traits: total seed anthocyanin content and seed coat colour. This makes sense because anthocyanin is a pigment that is mainly stored in the seed coat [15] . Cluster 2 on Chr13 contains QTLs regulating typical traits that differentiate wild from cultivated soybeans: trailing growth, pod number per plant and seed number per plant [16] . The trailing growth character of wild soybean results in a relatively longer overall growth period, which may lead to higher number of pods and more seeds per plant. The location of this cluster does not overlap with the previously identified QTL for indeterminate growth [17] . Cluster 3 on Chr19 contains QTLs that control pod colour and total seed antioxidant content. The close relationship between pod colour and total seed antioxidant content can be explained by two possible scenarios: (i) the pathway controlling the accumulation of pod colour pigmentation is also involved in the accumulation of seed antioxidants; or (ii) the genes controlling the two traits are incidentally located in close proximity. Identifying a possible causal gene for salt tolerance We focus our subsequent analyses on the salt tolerance locus we have identified in W05, which exhibits a much higher salt tolerance as compared with that of C08 ( Fig. 2a ). We find that salt tolerance is a dominant trait in our population. We identify a salt tolerance locus from W05 that spans a genomic region of 978 Kb and overlaps with the previously reported Ncl locus [18] , [19] , [20] , [21] . To better define this locus, we screen the remaining RI population and obtain two extreme groups (85 tolerant and 73 sensitive). Recombinant breakpoint analyses of the two groups using simple sequence repeat and SNP markers reduce the salt tolerance locus to a 388-Kb region on Chr03, which contains 43 predicted genes based on the annotated Williams 82 genome ( Fig. 2b ). Figure 2: Identification of a putative causal gene in the salt tolerance locus. ( a ) W05 exhibits a higher salt tolerance than C08. Bottom photos: primary leaves. ( b ) A 978-Kb salt tolerance locus is first identified by LOD score (upper panel), and narrowed down to a 388-Kb region using SNP and simple sequence repeat markers (middle panel) and extreme groups (lower panel). SL, sensitive line; TL, tolerant line. ( c ) W05 accumulates less Na + in the leaves than C08 72 h after NaCl treatment. N =4. Error bars=s.e.m., P <0.05. ( d ) Gene structure of GmCHX1 in W05 and Williams 82. Arrows indicate primer positions for insertion and real-time PCR studies. FW, fresh weight. Full size image When soybean plants are subjected to NaCl treatment, the Na + content and Na + /K + ratio in leaves are significantly lower in W05 compared with C08 ( Fig. 2c ), suggesting that ion transporters has an important role in salt tolerance. BLAST analysis of the 43 predicted genes reveals two genes ( Glyma03g32890 and Glyma03g32900 ) that have a high degree of similarity to cation H + exchangers ( CHX s) [22] . This 388-Kb region on Chr03 also has a duplicated segment on Chr19, likely a result of the past whole-genome duplication, but it does not possess a salt tolerance QTL. The two CHX genes present in the QTL on Chr03 are either absent or truncated in the duplicated segment on Chr19. Using the de novo sequencing data of W05, we identify a single scaffold containing the corresponding 388-Kb genomic region. Comparison of the genomic sequences of W05 and Williams 82 shows that Williams 82 had a Ty1/copia retrotransposon [23] inserted into exon 3 of the cation H + exchanger gene Glyma03g32900 , but not in its counterpart Glysoja01g005509 in W05 ( Fig. 2d ). PCR amplification and Sanger sequencing verify that the salt-sensitive parent C08 also contains the same insertion as Williams 82 ( Supplementary Fig. 6a ). 3′-RACE experiments show that Glysoja01g005509 in C08 produces a truncated transcript (encoding only 376 amino-acid residues versus 811 residues in the full-length Glysoja01g005509 in W05) ( Fig. 3a ). The salt-sensitive C08 appears to possess a loss-of-function variant of Glysoja01g005509 while real-time PCR analyses reveal that Glysoja01g005509 in W05 expresses a full-length transcript that is root specific ( Supplementary Fig. 6b ). Figure 3: The GmCHX1 gene is conserved among salt-tolerant soybean germplasms. ( a ) Structural variations in the GmCHX1 coding region of salt-sensitive germplasms, with salt-tolerant W05 as comparison. ( b ) SNP analyses and multiple amino-acid sequence alignments of the GmCHX1 coding region from different soybean germplasms. X denotes ambiguous amino acid due to low coverage of re-sequencing data. Black indicates conserved residues. ( c ) SNP analyses and multiple alignments of a 2-Kb promoter region of GmCHX1 from different soybean germplasms. Conserved bases are highlighted in black. R=G/A, Y=T/C. ( d ) Expression study of GmCHX1 in soybean germplasms. Real-time PCR of the GmCHX1 gene using primers specific to regions upstream (upper panel; for tolerant lines and C08) or downstream (lower panel; for all germplasms) referenced to the retrotransposon insertion site in C08, using RNA from salt-tolerant (green bars) and salt-sensitive germplasms (blue bars). N =3. Error bar=s.e.m. Full size image Phylogenetic analyses comparing Glysoja01g005509 to other monovalent cation/proton antiporters (CPA) that use monovalent ions as their substrate [22] ( Supplementary Fig. 7 ) show that the predicted gene product of Glysoja01g005509 belongs to the CHX clade of this superfamily. We name Glysoja01g005509 GmCHX1 to reflect its putative function. GmCHX1 is a potential salt tolerance determinant in soybean To further correlate the GmCHX1 gene with salt tolerance, we analyse 23 previously re-sequenced soybean accessions (12 salt-tolerant; 11 salt-sensitive) [2] . The SNPs in the coding region of GmCHX1 of the tolerant group, including W05, are conserved, whereas those of the sensitive group show varied genotypes ( Fig. 3a,b ). This difference is unique to only GmCHX1 within the entire 388-Kb region, supporting the claim that GmCHX1 is a putative causal gene for salt tolerance. More specifically, in the sensitive group, cultivated accessions C08 and C27 carry the same Ty1/copia retrotransposon as Williams 82 ( Supplementary Fig. 8 ), and wild salt-sensitive accessions (W06, W07, W08 and W09) have at least two types of deletions in their GmCHX1 exons ( Fig. 3a ). All SNPs within a 2-Kb promoter region of GmCHX1 are highly conserved in the tolerant accessions, but are varied among the sensitive accessions ( Fig. 3c ). Real-time PCR data show that all the sensitive accessions analysed produce undetectable or very low levels of full-length GmCHX1 transcripts as compared with the tolerant accessions ( Fig. 3d and Supplementary Fig. 9 ). Therefore, the GmCHX1 gene in the sensitive accessions is either non-functional or is expressed at very low levels. Rapid gain-of-function tests of GmCHX1 To further validate that GmCHX1 is a salt tolerance determinant in W05 and other salt-tolerant accessions tested, we perform a gain-of-function test by expressing the GmCHX1 cDNA from W05 in the hairy root culture of C08. Expression of the transgene is confirmed by real-time PCR ( Fig. 4c ). In the absence of NaCl treatment, both root cultures transformed with either GmCHX1 or green fluorescent protein ( GFP ; control) give healthy hairy roots ( Fig. 4a ). However, when subjected to NaCl treatments, roots transformed with GmCHX1 show significantly higher root fresh weights than the control ( Fig. 4b ), demonstrating that GmCHX1 from the major salt tolerance locus in W05 can alleviate salt stress. 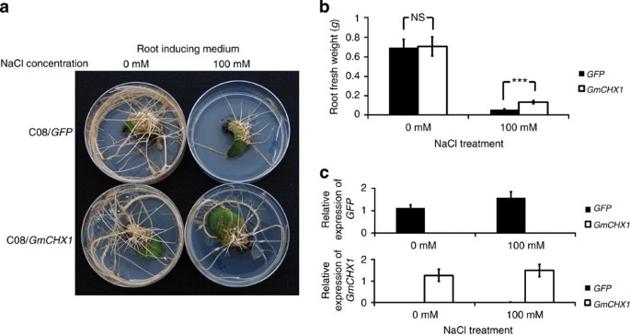Figure 4: Gain-of-function analysis ofGmCHX1using the hairy root system. (a) Phenotypes of transgenic hairy roots expressing eitherGFPorGmCHX1with or without NaCl treatment. Photos were taken 2 weeks after treatment. (b) Fresh weight of hairy roots with or without NaCl treatment.N≥12. Error bars, s.e.m. Data were analysed using Student’st-test. NS, not significant. ***P<0.001. (c) Expression of transgenes validated by real-time PCR. Upper panel:GFP; lower panel:GmCHX1.N≥12. Error bars=s.e.m. Figure 4: Gain-of-function analysis of GmCHX1 using the hairy root system. ( a ) Phenotypes of transgenic hairy roots expressing either GFP or GmCHX1 with or without NaCl treatment. Photos were taken 2 weeks after treatment. ( b ) Fresh weight of hairy roots with or without NaCl treatment. N ≥12. Error bars, s.e.m. Data were analysed using Student’s t -test. NS, not significant. *** P <0.001. ( c ) Expression of transgenes validated by real-time PCR. Upper panel: GFP ; lower panel: GmCHX1 . N ≥12. Error bars=s.e.m. Full size image We further confirm the function of GmCHX1 using transgenic tobacco BY-2 cells. Consistent with the hairy root assay, transgenic BY-2 cells ectopically expressing GmCHX1 show a higher survival rate under the treatment with 100 mM NaCl compared with the untransformed wild-type and the GFP transgenic control ( Fig. 5a,b ). Moreover, the GmCHX1 transgenic lines also maintain a lower Na + /K + ratio under salt stress ( Fig. 5c ), supporting our hypothesis that GmCHX1 is involved in ion homeostasis. 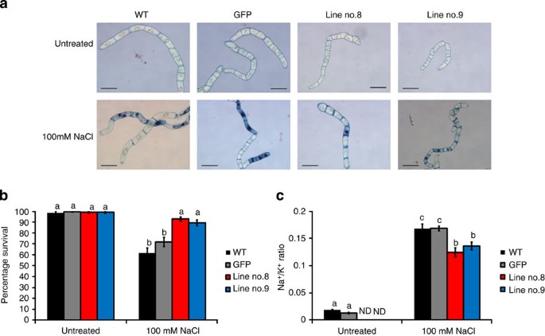Figure 5: Gain-of-function analysis ofGmCHX1using transgenic tobacco BY-2 cells. (a) Trypan blue staining of tobacco BY-2 cells under NaCl treatment. Four-day-old cells were treated with 100 mM NaCl or remained untreated in MS medium for 20 h before staining with Trypan blue. Nuclei of dead cells were stained blue. Scale bars, 100 μm. (b) Calculated survival rate based on the results of Trypan blue staining. The data were calculated from 14 randomly taken photos for each sample. (c) Na+/K+ratio of BY-2 cells under NaCl treatment. BY-2 cells were treated with 100 mM NaCl or remained untreated in MS medium for 4 h. Ion contents were determined using atomic absorption spectrophotometry.N=4. ND, non-detectable due to low signals. Numerical data inbandcwere analysed using one-way analysis of variance followed by the Tukey’spost hoctest (P<0.05). Error bars=s.e.m. Line no. 8 and Line no. 9 are two independent transgenic lines ofGmCHX1. WT, untransformed wild type; and GFP, BY-2 cells transformed with theGFPgene as a negative control. Figure 5: Gain-of-function analysis of GmCHX1 using transgenic tobacco BY-2 cells. ( a ) Trypan blue staining of tobacco BY-2 cells under NaCl treatment. Four-day-old cells were treated with 100 mM NaCl or remained untreated in MS medium for 20 h before staining with Trypan blue. Nuclei of dead cells were stained blue. Scale bars, 100 μm. ( b ) Calculated survival rate based on the results of Trypan blue staining. The data were calculated from 14 randomly taken photos for each sample. ( c ) Na + /K + ratio of BY-2 cells under NaCl treatment. BY-2 cells were treated with 100 mM NaCl or remained untreated in MS medium for 4 h. Ion contents were determined using atomic absorption spectrophotometry. N =4. ND, non-detectable due to low signals. Numerical data in b and c were analysed using one-way analysis of variance followed by the Tukey’s post hoc test ( P <0.05). Error bars=s.e.m. Line no. 8 and Line no. 9 are two independent transgenic lines of GmCHX1 . WT, untransformed wild type; and GFP, BY-2 cells transformed with the GFP gene as a negative control. Full size image One important goal of genomic and genetic studies of crop plants is to identify important loci and genes using unique germplasm resources, such as wild accessions, that can be used to improve agronomic traits and thereby agricultural productivity. Wild soybeans, in particular, are valuable genetic resources for improving soybean cultivation, owing to the rich collection and high genomic diversity of wild soybeans [1] , [2] , [7] , the absence of sexual reproduction barrier between wild and cultivated soybeans, and the availability of a reference genome [8] and SNP information [2] . In this study, we further explore the wild soybean genome by performing de novo genome sequencing of a wild soybean accession (W05) that has been shown to be genetically distinct from the cultivated model soybean Williams 82 (ref. 2 ). A de novo genome can facilitate the identification of genetic materials from wild soybean for crop improvement because comparing de novo genomes is more effective in identifying small and large structural variations between genomes [24] , [25] . To perform genetic analysis, we construct an RI population resulting from a cross between the de novo -sequenced W05 and the re-sequenced cultivated soybean accession C08 (ref. 2 ), a close relative of Williams 82. By adopting the bin map strategy [26] via re-sequencing of a core panel of the RI lines, together with phenotypic analyses of the core panel, we complete the mapping of major QTLs that regulate important agronomic traits such as nutritional quality, yield and stress tolerance. The genomic spans of most identified QTLs are narrow enough for use in marker-assisted breeding. Correlation studies of different QTLs also reveal potential interesting relationships among different traits. For example, the QTL for seed anthocyanin content does not overlap with the major QTL for seed antioxidant content, thus disproving anthocyanin as the most important antioxidant in seeds. Furthermore, the QTL of the trailing growth character overlaps the QTLs for pod number per plant and seed number per plant. The higher pod number and seed number per plant in wild soybeans are likely a result of the trailing growth. These traits are important for wild soybeans to survive in the natural environment by expanding their territories. However, human selection might have removed the trailing growth character in cultivated soybeans to ease the harvesting process and to increase crop density per unit area. Salinization poses a severe threat to agricultural productivity, affecting more than 20% of irrigated lands globally [27] . The wild soybean accession W05 exhibits a high tolerance towards salt stress and hence is a good genetic resource for improving salt tolerance in soybean. By exhausting the lines in our RI population for QTL mapping and extreme group study, we have identified a 388-Kb major salt tolerance locus in the soybean genome. The exceptionally long linkage disequilibrium of the soybean genome [2] has posed a major obstacle in finding causal genes in a QTL. To identify the causal gene for salt tolerance within the 388-Kb region, we make use of a combination of genomic information and physiological data. The lower Na + distribution in the leaves of the salt-tolerant line W05 compared with that in the salt-sensitive C08 has drawn our attention to ion transporter genes. By comparing the de novo genome sequencing data of the wild accession W05 to those of C08 and the reference genome Williams 82, we reveal the presence of a retrotransposon insertion in the ion transporter gene GmCHX1 of the salt-sensitive C08 and Williams 82, whereas the salt-tolerant W05 retains an intact GmCHX1 sequence. This kind of structural variation is hard to be detected without de novo sequencing data. Whole-genome-re-sequencing data are used to examine the changes in the gene structure of GmCHX1 in genetically unrelated germplasms to validate the correlation between salt sensitivity and loss-of-function or low gene expression of GmCHX1 . The gain-of-function tests have finally shown that GmCHX1 can confer salt tolerance, probably via lowering of the Na + /K + ratio. Interestingly, the leaves of the salt-tolerant W05 also exhibit a lower Na + /K + ratio than the salt-sensitive C08. It appears that the functional GmCHX1 gene is an ancestral trait and the sensitive accessions have accumulated different types of mutations either in the coding region (eliminating/reducing the gene function) or the promoter region (lowering the expression). At this point, we cannot completely eliminate the possibility that the causative mutation might involve small RNA regulation or control by an adjacent transcription factor gene. However, these possibilities are less likely, given that the only annotated transcription factor gene located within the 388-Kb region does not exhibit a major sequence difference between tolerant and sensitive parents. The elimination of GmCHX1 in salt-sensitive germplasms may be an example of negative selection against a stress tolerance gene in unstressed environments. The expression of stress tolerance genes can be an energy burden on the plant if the functions of these genes are not required. Although it has long been believed that Cl − homeostasis has a critical role in soybean salt tolerance [28] , [29] , [30] , accumulated evidence shows that cation transporters are major salt tolerance determinants in plants. For example, high-affinity potassium transporters, which unload Na + from the root xylem, reduce Na + accumulation in the leaves of important crops such as rice and wheat [31] , [32] . The CPAs constitute another important superfamily of ion transporters, which can be further divided into two clades: CPA1 and CPA2 (ref. 22 ). Members of the CPA1 subfamily such as Salt Overly Sensitive 1 (SOS1) and Na + /H + antiporters 1 (NHX1), which are localized on the plasma membrane and tonoplast, respectively, can protect plants by excluding or compartmentalizing Na + (refs 33 , 34 ). The possible functions of NHX homologues isolated from soybean have also been reported [35] . CHXs are members of the CPA2 subfamily whose protective functions remain largely unclear. A few studies using other plant models implicate that some CHXs may be involved in Na + transportation and salt tolerance [36] , [37] , [38] . Here we provide gain-of-function data to confirm that the GmCHX1 gene identified by our genomic and genetic studies confers salt tolerance. In summary, we have developed an efficient strategy using a combination of different whole-genome-sequencing approaches that can greatly enhance the efficiency of uncovering QTLs and genes for beneficial traits in crop breeding. By using the de novo sequencing data of a wild soybean genome and the re-sequencing data of soybean germplasms, we are able to identify a candidate causal gene for salt tolerance, validated via gain-of-function tests. In addition, the sequence information on the 868-Mb de novo -assembled wild soybean genome and the mapping of 15 major QTLs resulting from this work will also benefit soybean researchers and breeders for further mining of the wild soybean genome. W05 de novo sequencing and assembly Eight libraries of different insertion sizes (180, 260, 326, 817, 2, 2.3, 6 and 10 Kb) were sequenced using the Illumina GAII platform. Raw reads were filtered to eliminate sequencing errors, by removing reads with N or polyA for >10% of bases, low quality reads (reads from short insert-size libraries of 180–817 bp: with 50 or more bases having Phred-scaled quality score (Q-score) lower than or equal to 7; reads from large insert-size libraries of 2–10 Kb: with 15 or more bases having Q-score lower than or equal to 7), reads contaminated with adapter sequence (with >10 bp aligned to the adapter, allowing three mismatches at most), reads with wrong insertion size either due to paired or overlapping reads, and reads identical in both ends resulting from PCR amplification. The minimum average Q-score for each library is Q20 after trimming. After data pre-processing, we obtained a total of 73.5 Gb clean reads. SOAPdenovo [9] was used to perform genome assembly. Clean data from small insert-size libraries were used to construct contigs, with K-mer set to 35 bp, and clean data from large insert-size libraries were used to connect contigs to form scaffolds according to the pair-end relationship. The scaffold gaps were then filled, with scaffolds of 200 bp or below being discarded from the final version. Repeat and non-coding RNA annotation To annotate the transposable elements in the wild genome, de novo and homology prediction were applied. For the de novo annotation, RepeatModeler (part of RepeatMasker) and LTR_FINDER [39] were used to identify the de novo repeats to build a library for transposable elements. The de novo -based repeat library, soyTEdb [23] , and Repbase [40] library were then used to identify the repeats by homology using RepeatMasker. To annotate the tandem repeats, Tandem Repeat Finder [41] and RepeatMasker (parameter ‘-noint’, http://www.repeatmasker.org , version 3.2.9) were used. To annotate the protein-coding transposable elements, RepeatProteinMask (part of RepeatMasker) was used to search the repeat-related proteins against the transposable element protein database ( http://www.repeatmasker.org/RepeatProteinMask.html#database ). tRNAscan-SE [42] and INFERNAL [43] were used to predict non-coding RNAs within the wild soybean genome using parameters for eukaryotic species. Pseudo-tRNA and tRNA genes overlapping with SINE repeat regions were discarded. To identify ribosomal RNA fragments, Blastn ( E -value=1e −5 , aligned length ≥50 bp) was used to align potential ribosomal sequences with plant ribosomal RNAs. Both microRNA and small nuclear RNA genes were predicted by INFERNAL against the Rfam database [43] . Gene model prediction and annotation De novo gene prediction, homology prediction and transcript sequence-based annotation were used to identify protein-coding genes. Augustus (version 2.5.5; ref. 44 ) and Glimmer-HMM (version 3.0.1; ref. 45 ) were used in the de novo gene prediction using the repeat masked scaffold sequence based on the HMM model, with parameters trained for Arabidopsis thaliana . Homologous proteins from related species were mapped to the genome using BLAST (version 2.2.23, E -value cutoff set at 1e −5 ). Aligned sequences as well as its query proteins were filtered, and GeneWise (version 2.2.0; ref. 46 ) was then used for searching accurately spliced alignments. EST sequences of G. max and G. soja (from NCBI) were aligned to scaffolds using BLAT (version 34, G. max : identity >0.93, coverage >0.8; G. soja : identity >0.95, coverage 0.8) to generate fragmental alignments. These alignments were linked together using PASA according to sequence overlaps [47] . RNA-Seq data were generated using three cDNA libraries (insertion size 200 bp) constructed from the total RNA of trifoliate and primary leaves, and roots of young seedlings of W05, and were sequenced with Illumina GAII to produce PE reads (75 bp for each read). A total of 7.5 Gb of data were produced. RNA-Seq data from W05 were aligned to scaffolds using TopHat [48] to identify candidate exon regions. The donors and acceptors at the splicing sites were then identified. Finally, the transcripts were assembled using Cufflinks (version 2.1.1; ref. 48 ) for the EST and RNA-Seq data, which make up the third gene set. GLEAN [49] was then used to integrate all three gene predictions ( de novo , homology-based and transcript-based) into a consensus gene set. Gene functions were assigned according to the best match of the alignments using Blastp to the SwissProt and TrEMBL databases (Uniprot release 2012_03). Motifs and domains were determined by InterProScan (version 4.7) against protein databases including ProDom, PRINTS, Pfam, SMART, PANTHER and PROSITE. Gene Ontology IDs were obtained from the corresponding InterPro entries. This Gene Ontology category was compared with that of the published Williams 82 annotation ( Supplementary Fig. 3 ). All genes were aligned against the Kyoto Encyclopedia of Genes and Genomes (KEGG) database (release 58) and the pathways in which the genes might be involved were derived from the matched genes in KEGG. To independently validate the annotation, the transcriptome sequencing data were assembled using Trinity r2013-02-25 with a minimum contig length of 200 (ref. 10 ). TransDecoder ( http://transdecoder.sourceforge.net/ ) was used to extract best protein-coding regions from the Trinity transcripts. Trinity contigs were mapped to the annotated genome using the following parameters: (i) E -value=1e −50 ; (ii) identity >0.9; and (iii) the transcripts can be longer than the annotated sequence, but cannot be shorter than the annotated sequence by 100 bp. CEGMA (v2.4.010312) was used to access the genome completeness [11] . RI population construction and phenotype recording The wild parental line W05 originated in Henan Province in China and the cultivated soybean C08 was a close relative of Williams 82 from USA ( http://wildsoydb.org/strains/soybean ). W05 and C08 were reciprocally crossed to obtain F1 seeds. F1 plants were self-pollinated to obtain F2 seeds. Single-seed descendants were propagated from F2 to F7 to obtain a RI population consisting of 455 independent lines. Some segregants at higher generations were collected because of differences in agronomic traits, making a total RI population of 552 lines. Starting from F8, mixed seeds were collected and propagated for each line. A core panel of 96 RI lines that exhibited a diverse spectrum of growth period duration was selected for sequencing and mapping analyses. Eighteen phenotypic traits of this population were recorded in a greenhouse (22°25′7″ N, 114°12′26″ E) or in open fields in an experimental farm (38° 35′0″ N, 116° 48′0″ E) from 2008 to 2012. Detailed descriptions of the measurement method for each trait are provided in Supplementary Table 10 . Population re-sequencing and SNP identification The HiSeq 2000 sequencing platform was used to generate 1.24 G 75-mer pair-end reads of the selected core panel of 96 RI lines, with an average of 12.9 M reads for each RI line. Properly paired and uniquely mapped reads were then used to call SNPs. Reads containing >10 Ns were filtered before alignment. SOAP2 (ref. 50 ) was used to map filtered reads back to the Williams 82 genome using the following parameters: seed length of 32 bp, maximum three mismatches allowed in each read, minimum aligned length of 35 bp to identify a mapped read. Reads that could not be properly paired or resulted in multiple alignment sites were discarded. SNPs of the population were called by SAMtools [51] with the following parameters: base quality of the SNP site no <30 and no >3 SNPs in any 10 bp window along the reference genome. Filtered SNPs were used to calculate the heterozygosity of each RI line using H=((no. of heterozygous SNPs)/(no. of total SNPs)) × 100%. Genotyping and QTL identification The SNPs were further filtered by the following criteria: SNPs were of the two parental genotypes and homozygous, and there were at least 20 RI lines with SNPs at a single site. The maximum parsimonious inference of recombination package was adopted to identify recombinant breakpoints and generate bins. The R/qtl package was used to calculate the genetic distance between markers in Kosambi mapping function [13] . A recombinant hot spot was identified between Chr13 (physical position from 20,343,655 to 33,600,100 bp) and Chr11 (physical position from 23,866,522 to 39,171,759 bp) based on pair-wise recombination fractions and LOD scores ( Supplementary Fig. 10 ). QTLs were identified using QTLCartographer ( http://statgen.ncsu.edu/qtlcart/ ). Interval mapping and composite interval mapping were performed for each data set with a 10-cM scanning window and a 0.5-cM walking step. For the identification of major QTLs, the LOD score cutoff was determined by 1,000 times permutation at P =0.05. The boundary of each major QTL was then defined by a LOD score-drop of 1.5 (ref. 52 ). The correlation between different phenotypes was calculated using the Predictive Analytics Suite Workstation Statistics (PASW Statistics 18.0.0). NaCl treatments and ion content analyses of soybean plants Soybean seeds were germinated in a greenhouse on vermiculite. When the primary leaf appeared, the seedlings were transferred to a hydroponic system with half-strength Hoagland’s solution for 5 days. Salt treatment was applied by replacing the growth solution with fresh half-strength Hoagland’s solution containing 0.9% NaCl (or no NaCl for the untreated control). For phenotype observations, the seedlings were treated for 6 days. For ion content analyses, tissues were collected at 24 or 72 h after treatment and ground in 1% acetic acid for soluble ion extraction. Na + and K + ion contents were analysed using the flame atomic absorption spectrophotometer (Hitachi Z2300) according to the manufacturer’s instructions. Fine mapping of salt tolerance locus Primers for SNP genotyping were designed based on the re-sequencing data [2] and the Williams 82 reference genome [8] using the ARMS-tetra primer method with the BatchPrimer3 programme [53] . A list of primers used can be found in Supplementary Data 2 . PCR was conducted in a 15-μl reaction mixture containing 1 × buffer, 3 mM MgCl 2 , 0.2 mM dNTPs, 0.3 μM of each primer, 100 ng genomic DNA template and 0.5 U GoTaq DNA polymerase (Promega Corp., Fitchburg). The thermal cycler was programmed with an initial 2 min at 94 °C, followed by 35 cycles of 30 s at 94 °C, 30 s at the primer-specific annealing temperature and for a marker-specific extension time at 72 °C ( Supplementary Data 2 ). After the thermal cycles, an additional 10 min at 72 °C was added to allow for the completion of extension. PCR products were resolved on 2% agarose gel in 1 × TAE buffer. Analyses of GmCHX1 structural variations The consensus sequences of GmCHX1 in different soybean germplasms were from previous mapping results [2] , with reference to the genomic coordinates of Williams 82, and were then translated into amino-acid sequences. Differences among the consensus sequences were examined after alignment by the ClustalW2 programme [54] . Retrotransposon insertions in the GmCHX1 gene were amplified from genomic DNA and detected using PCR ( Supplementary Figs 6 and 8 ). The Sanger method was used to confirm the sequence of the coding region of GmCHX1 in different germplasms (tolerant: C01, C14, W01–W05 and W11; sensitive: C08, C12 and W06–W10). Cloning and gene expression of GmCHX1 The cDNA of GmCHX1 was obtained from total RNA extracted from the root. 3′ RACE was performed using the SMARTer RACE cDNA Amplification Kit (Clontech, cat. no. 634923, CA) according to the manufacturer’s instructions. Real-time PCR was conducted using the One Step SYBR PrimeScript RT-PCR Kit II (TaKaRa Biotechnology Co. Ltd, Dalian, China) according to the manufacturer’s instruction, with a reaction volume of 20 μl containing 100 ng total RNA, using the CFX96 Touch Real-Time PCR Detection System (Bio-Rad, Hercules). Primers for real-time PCR were listed in Supplementary Data 2 . The relative expression of target genes was calculated using the 2 −ΔΔ C t method [55] . Gain-of-function test of GmCHX1 in hairy root system The full-length coding sequence of GmCHX1 from W05 was cloned into the binary vector V7 (ref. 56 ) between Xba I and Xho I sites downstream of the constitutive Cauliflower Mosaic Virus 35S promoter. As a negative control, the gene for the GFP was cloned instead of GmCHX1 using the same vector and promoter. Both constructs were then transformed into the salt-sensitive parent C08. The soybean hairy root transformation and salt treatments were performed as previously described [57] with some modifications. Surface-sterilized soybean seeds were germinated on germination medium (15 mg l −1 NaH 2 PO 4 ·H 2 O, 1 mM CaCl 2 ·2H 2 O, 25 mM KNO 3 , 1 mM (NH 4 ) 2 SO 4 , 1 mM MgSO 4 ·7H 2 O, 0.1 mM Na 2 EDTA·2H 2 O, 0.1 mM FeSO 4 ·7H 2 O, 10 mg l −1 MnSO 4 ·2H 2 O, 2 mg l −1 ZnSO 4 ·7H 2 O, 3 mg l −1 H 3 BO 3 , 0.25 mg l −1 Na 2 MoSO 4 ·2H 2 O, 0.025 mg l −1 CuSO 4 ·5H 2 O, 0.025 mg l −1 CoCl 2 ·6H 2 O, 0.75 mg l −1 KI, 1 × B5 vitamin (10 mg l −1 thiamine, 1 mg l −1 pyridoxal phosphate, 1 mg l −1 nicotinic acid and 100 mg l −1 myo-inositol), 2% sucrose, 0.6% agar, pH 5.8) for 4 days (16 h light/8 h dark). Agrobacterium rhizogenes strain K599 containing the recombinant constructs was grown in yeast extract peptone medium containing 50 mg l −1 kanamycin and 200 μM acetosyringone at 28 °C for 16 h. It was then used to infect the cotyledons through scalpel incisions. The cotyledons were co-cultivated with A. rhizogenes in the dark for 5 days on moist filter paper. After that, the infected cotyledons were transferred to root-inducing medium (4.3 g l −1 Murashige and Skoog (MS) medium, 1 × B5 vitamin, 3% sucrose, 250 mg l −1 cefotaxime and 50 mg l −1 kanamycin). After 2 weeks, cotyledons with roots emerging from the incision sites were transferred to new root-inducing medium with 100 mM NaCl or medium without NaCl as untreated control. Root mass was weighed about 2 weeks after treatment. Gain-of-function test of GmCHX1 in transgenic tobacco BY-2 cells The same recombinant constructs used in the hairy root system described above were used to transform tobacco BY-2 cells using A. tumefaciens strain LBA4404. For Trypan blue staining, 4-day-old BY-2 cells were suspended in MS medium with or without 100 mM NaCl for 20 h. Cells were stained with Trypan blue (Sigma, cat. no. T8154) for 5 min before being observed under the microscope (Nikon E80i). To determine ion contents, 25 ml 4-day-old BY-2 cells were mixed with 25 ml MS medium with or without 200 mM NaCl (to make up to a final concentration of 100 mM) for 4 h. The cells were harvested and washed with 100 ml deionized water by suction filtration. Cells were microwaved for 10 s in 5 ml 1% acetic acid at 1,100 W three times. Cell lysates were then centrifuged at 13,000 g for 10 min and subjected to ion content analysis. Statistical analyses The effects of salt treatment on Na + accumulation in the leaves of W05 and C08, the survival rate and ion content of tobacco BY-2 cells under NaCl treatment were analysed using a one-way analysis of variance followed by the Tukey’s post hoc test at P <0.05. The effects of salt treatment on the root fresh weight of C08 ectopically expressing GmCHX1 from W05 or GFP were analysed using the Student’s t -test. Accession codes: Full-length coding sequences of GmCHX1 for W05 and C08 have been deposited in GenBank/EMBL/DDBJ nucleotide core database under the accession codes KF879911 and KF879912, respectively. Genome and transcriptome sequencing data of W05 have been deposited in GenBank/EMBL/DDBJ Sequence Read Archive under the accession codes SRR1185929 to SRR1185926 and SRR1185321 to SRR1185323 , respectively. Genome sequence data for W05 have been deposited in GenBank/EMBL/DDBJ nucleotide core database under the accession code AZNC00000000 . How to cite this article: Qi, X. et al. Identification of a novel salt tolerance gene in wild soybean by whole-genome sequencing. Nat. Commun. 5:4340 doi: 10.1038/ncomms5340 (2014).